Manifestation of magnetic quantum fluctuations in the dielectric properties of a multiferroic Insulating magnets can display novel signatures of quantum fluctuations as similar to the case of metallic magnets. However, their weak spin-lattice coupling has made such observations challenging. Here we find that antiferromagnetic (AF) quantum fluctuations manifest in the dielectric properties of multiferroic Ba 2 CoGe 2 O 7 , where a ferroelectric polarization develops concomitant to an AF ordering. Upon application of a magnetic field ( H ), dielectric constant shows a characteristic power-law dependence near absolute zero temperature and close to the critical field H c =37.1 T due to enhanced AF quantum fluctuations. When H > H c , the dielectric constant shows the temperature-dependent anomalies that reflect a crossover from a field-tuned quantum critical to a gapped spin-polarized state. We uncover theoretically that a linear relation between AF susceptibility and dielectric constant stems from the generic magnetoelectric coupling and directly explains the experimental findings, opening a new pathway for studying quantum criticality in condensed matter. Quantum phase transitions (QPT) in correlated electron materials have been intensively studied in recent years in an effort to understand quantum critical phenomena and exotic order realized near a quantum critical point (QCP) [1] . The Fermi-liquid state of the conduction electrons shows instabilities near a magnetic QCP, often leading to non-Fermi-liquid behaviour and even exotic superconductivity [2] , [3] . In the absence of conduction electrons, a magnetic QCP has been found in Ising ferromagnets by applying a transverse magnetic field [4] , [5] and in spin-dimer compounds that show Bose–Einstein Condensation (BEC) [6] , [7] , [8] . QPT can also be found in ferroelectric (FE) materials where the electric polarization ( P ) serves as the order parameter. An archetypical case is SrTiO 3 , in which a huge dielectric constant ( ε >10 4 ) is observed at low temperatures ( T ) without showing any long-range order due to quantum fluctuations in the vicinity of a FE QCP [9] , [10] , [11] . Substituting 16 O with 18 O as well as applying external pressure have also been shown to be effective ways to control the FE transition temperature [12] , [13] . Recently, multiferroic materials have been intensively studied due to their potential as possible components of multifunctional devices [14] , [15] , [16] , [17] , [18] , [19] . Moreover, efforts to understand the general mechanisms of cross-coupling between magnetism and ferroelectricity have made great progress in the fundamental science of competing magnetic interactions and spin-orbit coupling in various complex materials [20] , [21] . Quantum critical phenomena in these materials are also of great interest, because one may study the critical behaviours of coupled ferroic order parameters in the quantum critical regime possibly due to their rather strong spin-lattice coupling. In general, even in multiferroic materials, it is still difficult to directly observe quantum fluctuations of the antiferromagnetic (AF) order parameter by probing the dielectric properties. This is because the dielectric properties are often determined by low energy fluctuations near the center of the Brillouin zone (uniform response). Moreover, in most multiferroics with magnetically induced ferroelectricity, frustrated spin interactions are present so that the magnetic field often induces a first-order transition between different spin structures and related FE phases. Furthermore, due to rather a large exchange interaction among spins, the magnetic field required to induce such a phase transition can easily surpass 100 T~10 meV. Thus far, the search for the non-classical properties in multiferroic materials is limited to a few cases in metal-organic materials [22] , [23] . In these systems, magnetic order sets in as a non-collinear arrangement of Cu 2+ spins with S =1/2, with small exchange energy and low magnetic ordering temperature ( T N <2 K). Moreover, they have rather weak magnetodielectric coupling (Δ ε / ε <3%) and small electric polarization ( P <30 nC m −2 ), which makes it challenging to study quantum critical phenomena through their dielectric properties. Crystals in the melilite group with magnetic ions ( A 2 BX 2 O 7 , A =Ca, Sr, Ba, B =Mn, Fe, Co, Cu and X =Si, Ge) turn out to have several features to overcome the above hurdles [24] , [25] , [26] , [27] . They exhibit a simple magnetic structure with minimal spin frustration and a relatively low ordering temperature. In this group, we choose to study Ba 2 CoGe 2 O 7 (BCGO), which has the largest electric polarization (~180 μC m −2 at 28 T). It is known to form a tetragonal and non-centrosymmetric structure (space group ) with two CoO 4 tetrahedra in a unit cell connected through GeO 4 tetrahedra in the ab -plane [28] ( Fig. 1a ). The alternating tilting angle ( κ ) of the CoO 4 tetrahedra along the diagonal direction within the ab -plane ( Fig. 1a ) plays a key role in the magnetoelectric (ME) coupling between the AF order parameter and the uniform electric polarization. The Co 2+ spins form simple square lattice layers and are antiferromagnetically coupled in the ab -plane below 6.7 K. The magnetic propagation vector is Q =(1,1,0) and corresponds to the AF layers that are ferromagnetically ordered along the c -axis [28] . The system has been known to possess an easy-plane anisotropy as confirmed by magnetic susceptibility ( Supplementary Fig. 1 ), inelastic neutron diffraction [28] , electron spin resonance and far infrared spectroscopy [29] . However, recent studies on the lattice and magnetic structure [30] , [31] show that BCGO actually has a lower symmetry with weak orthorhombic distortion in the plane and result in magnetic space group Cm ′ m 2′. 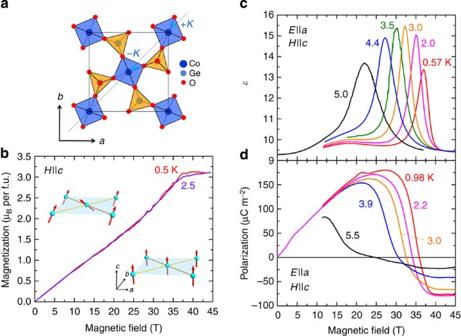Figure 1: Magnetic field-induced phase transition in multiferroic Ba2CoGe2O7. (a) Structure of Ba2CoGe2O7as perceived from a direction perpendicular to theab-plane. Two Co2+ions sit at the (0,0,0) and (0.5,0.5,0) positions of a unit cell. Co2+ions are placed inside a oxygen tetrahedra that is tilted from the [110] direction by angles +κand−κ. (b) Magnetization as a function of the magnetic field along thec-axis. Magnetization saturates aboveHc=37.1 T. Inset shows the canted spin structure atH<Hc(top left) and fully saturated spin structure atH≥Hc(bottom right). (c) Dielectric constant (ε) measured at 1 kHz. (d) Electric polarization (P) along thea-axis as a function of the magnetic field applied along thec-axis. Magnetic field-sweep rates forεandPmeasurements are 0.0083 and 0.033 T s−1, respectively. Figure 1: Magnetic field-induced phase transition in multiferroic Ba 2 CoGe 2 O 7 . ( a ) Structure of Ba 2 CoGe 2 O 7 as perceived from a direction perpendicular to the ab -plane. Two Co 2+ ions sit at the (0,0,0) and (0.5,0.5,0) positions of a unit cell. Co 2+ ions are placed inside a oxygen tetrahedra that is tilted from the [110] direction by angles + κ and− κ . ( b ) Magnetization as a function of the magnetic field along the c -axis. Magnetization saturates above H c =37.1 T. Inset shows the canted spin structure at H < H c (top left) and fully saturated spin structure at H ≥ H c (bottom right). ( c ) Dielectric constant ( ε ) measured at 1 kHz. ( d ) Electric polarization ( P ) along the a -axis as a function of the magnetic field applied along the c -axis. Magnetic field-sweep rates for ε and P measurements are 0.0083 and 0.033 T s −1 , respectively. Full size image A change in the FE polarization appears below the AF ordering temperature ( T N =6.7 K, Supplementary Fig. 1 ) [24] , [26] and originates from the p – d hybridization ( pd H) mechanism [32] , [33] , [34] . According to this mechanism, an electric polarization ( P ij ) develops along the bond direction e ij connecting the i -th spin, S i and the j -th ligand in the form Interestingly, the pd H mechanism does not originate from a frustrated spin structure such as a spiral or a ↑↑↓↓ spin structure, which spontaneously breaks spatial inversion symmetry upon magnetic ordering [14] , [17] , [19] , [35] . Instead, P is induced by a combination of spin-orbit interaction and anisotropic hybridization between the p - and d -orbitals of oxygen and the magnetic ion. We further note that the ME response of BCGO described above can be explained by following the general symmetry arguments without invoking any microscopic model at low fields [36] , [37] . Here we present experimental and theoretical study of the field-induced QPT in BCGO, around which the signatures of AF quantum fluctuations are reflected in its dielectric constant due to strong ME coupling. Our analysis based on a Ginzburg–Landau (GL) free energy shows that the dielectric constant of BCGO and the universality class of mean-field type emerges due to increased effective dimension at the putative QCP, being consistent with experimental results. Magnetic field-dependence of magnetization A QPT from AF to paramagnetic (PM) is realized in this system at high magnetic fields. In BCGO, spins are confined in the ab -plane with a simple AF configuration [28] . Sublattice magnetization ( L ) also lies in the ab -plane with weak ferromagnetic moment perpendicular to L at zero field. When H is applied along the c -axis, spins gradually rotate towards the c -axis and L decreases simultaneously. Finally, above H c , all the magnetic moments become nearly parallel to the c -axis. This scenario is supported by the magnetization curves M ( H ) measured for H ‖ c -axis and is shown in Fig. 1b . At 0.5 K, M increases monotonically up to a saturation value of ~3.1 μ B per f.u. above H c =37.1 T, which is consistent with full saturation of the S =3/2 spins. However, the signatures of the AF–PM phase transition are not so apparent in the M ( H ) curves because the order parameter is staggered, and M ( H ) is the response to a uniform field [38] . Magnetic phase transition observed by FE properties Counter-intuitively, the magnetic phase transition is clearly observed in the FE properties of BCGO due to a combination of two properties: (1) a strong ME coupling and the staggered tilting ( κ ) angle of the CoO 4 tetrahedra that allows coupling between the uniform polarization and (2) the staggered moment (order parameter). Figure 1c shows the ε ( H ) curves measured along the a -axis when H is applied along the c -axis. The AF transition is marked by the onset of a peak in ε (ref. 24 ). Upon cooling, the peak shifts to higher magnetic fields and eventually gets very close to H c at 0.57 K. The peak intensity increases concomitantly showing a large magnetodielectric effect of Δ ε / ε (0 T)~66 % at 3 K with a decrease upon further cooling. The field-induced shift of the AF transition is also reflected in the P ( H ) curves measured in the same configuration ( Fig. 1d ). P increases linearly in H at low fields (<15 T) [24] , reaches a maximum, and then decreases rapidly to reach a constant negative value above H c . The field value at which P decreases rapidly shifts to higher magnetic fields up to H c upon cooling thus indicating the suppression of the magnetically induced polarization. The magnetic field-dependence of P can be explained by the pd H mechanism. By calculating equation (1) explicitly for each inequivalent Co 2+ spin, the a -axis polarization has contributions from two Co 2+ sites [26] . where θ i , φ i are the spherical coordinates of the corresponding spins. Under a magnetic field applied along the c -axis, only the out-of-plane spin component (cos θ i ∝ M c ≡ M ) contributes to the electric polarization. Therefore, equation (2) can be rewritten as . This expression predicts P =0 when M is fully saturated to become M S , that is, L is suppressed to zero. However, P shows a finite negative value at H > H c in experiments ( Fig. 1d ). In addition, we found that the P ( H ) data shown in Fig. 1d could not be reversed by a negative poling procedure. To account for such negative P contribution, a slight tilting of magnetic field (<4° away from the c -axis), which can practically exist in high field experiments, should be considered. In such a situation, a small in-plane magnetization coming from a small in-plane field (<2.6 T) is likely to exist even above H c . Given that BCGO belongs to a non-centrosymmetric space group that allows piezoelectric coupling, the in-plane magnetization can naturally generate an additional in-plane P through the magnetostriction. Moreover, due to the pd H mechanism, the small tilting of magnetic field away from the c -axis can also induce additional P component perpendicular to the in-plane magnetization direction as demonstrated by Murakawa et al. [26] in a low field study. It can be simply shown that the additional in-plane P contribution from either the magnetostriction effect or the pd H mechanism should be roughly proportional to M 2 . Therefore, by adding the additional P term that is proportional to − M 2 to Equation (2), we can quantitatively explain the full P ( H ) curve in our experiments (see Supplementary Fig. 2 and Supplementary Note 1 for details). More evidence for a phase transition at high magnetic fields is provided by T -dependent measurements under constant H . 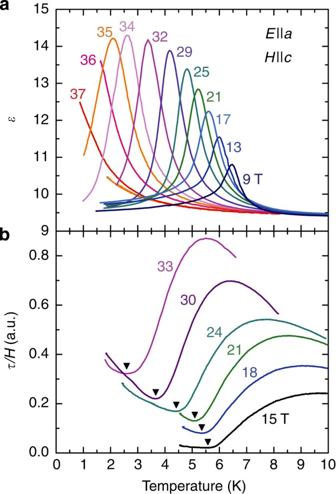Figure 2: Suppression of magnetic long-range order by magnetic field. (a) Dielectric constant and (b) magnetic torque normalized by the magnetic field (τ/H) as a function of temperature atH<Hc. For the torque measurements, the magnetic field was slightly canted away from thec-axis (~1°).τ/HversusTcurves are shifted for clarity. Minimum points (indicated by black triangles) inτ/HdenoteTN. Typical temperature sweep rate is 0.0167 K s−1. Figure 2a shows the T -dependence of ε under different magnetic fields below H c . A small peak appears at T N for low fields and grows while shifting to lower temperatures for increasing values of H . The peak saturates above 34 T, which is quantitatively consistent with the isothermal magnetic field-sweep measurements. Additional evidence for a thermodynamic phase transition is provided by the T -dependence of the magnetic torque ( τ / H , Fig. 2b ). The minima in τ / H denote values of T N that coincide with the peak positions of ε and further prove that ε is directly related to the AF order. The absence of hysteresis in the H - and T -dependence of ε suggests that the phase transition is continuous (see Supplementary Fig. 3 and Supplementary Note 2 for details). Figure 2: Suppression of magnetic long-range order by magnetic field. ( a ) Dielectric constant and ( b ) magnetic torque normalized by the magnetic field ( τ / H ) as a function of temperature at H < H c . For the torque measurements, the magnetic field was slightly canted away from the c -axis (~1°). τ / H versus T curves are shifted for clarity. Minimum points (indicated by black triangles) in τ / H denote T N . Typical temperature sweep rate is 0.0167 K s −1 . Full size image Gapped spin-polarized state above Remarkably, another energy scale is found through ε measurements when magnetic field is further increased above H c . 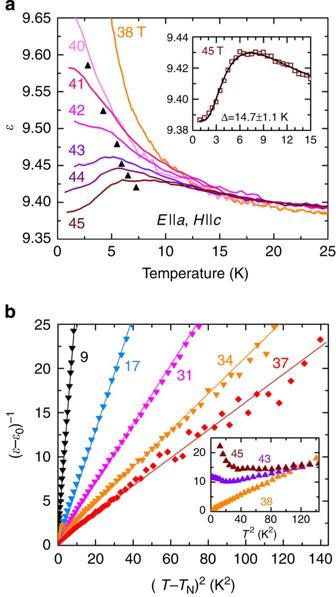Figure 3: Gapped spin-polarized state above the critical field andT2power-law behaviour in the dielectric constant. (a) Dielectric constant as a function of temperature above the saturation magnetic field. Black triangles point to anomalies inεthat appear above 40 T. Inset shows the expandedε(T) curve at 45 T, which show a sudden drop of ε below ~6.5 K. Dotted line is the fit to the equation with a spin gap with 14.7±1.1 K explained in text. (b) Inverse ofε−ε0as a function of (T−TN)2atH≤Hc. at constant magnetic fields (triangles, inverses triangles, and diamonds indicate magnetic field below, at, and above theHc). The linear behaviour in (ε−ε0)−1supports that theT2behaviour is robust within a wide magnetic field range up to 12 K aboveTN. Solid lines are guides for the eyes. Inset shows the same plot atH>Hc. TheT2behaviour is satisfied when the magnetic field is close toHc, but deviates quickly as an anomaly inεis observable at higher magnetic fields. Figure 3a shows ε ( T ) curves at a constant magnetic field for H > H c . At 39 T, ε increases monotonically on cooling because it is very close to the T =0 critical field H c . Notice that the ε ( T ) curves show the changes in slope at low temperatures at fields of 40 and 41 T. Strikingly, this feature becomes a shoulder at 42 T and ~5.2 K and evolves to a broad maximum when the magnetic field is further increased. These features, denoted as T * (indicated by filled triangles in Fig. 3a , see Supplementary Fig. 4 and Supplementary Note 3 for details), indicate the emergence of an energy scale that characterizes the gapped spin-polarized state. At 45 T, T * is found at ~7 K and ε ( T ) data can be fitted with an energy gap as (inset in Fig. 3a ). We note that this fit is not applicable to ε ( T ) data at lower magnetic fields, possibly due to a higher order background. Figure 3: Gapped spin-polarized state above the critical field and T 2 power-law behaviour in the dielectric constant. ( a ) Dielectric constant as a function of temperature above the saturation magnetic field. Black triangles point to anomalies in ε that appear above 40 T. Inset shows the expanded ε ( T ) curve at 45 T, which show a sudden drop of ε below ~6.5 K. Dotted line is the fit to the equation with a spin gap with 14.7±1.1 K explained in text. ( b ) Inverse of ε − ε 0 as a function of ( T − T N ) 2 at H ≤ H c . at constant magnetic fields (triangles, inverses triangles, and diamonds indicate magnetic field below, at, and above the H c ). The linear behaviour in ( ε − ε 0 ) −1 supports that the T 2 behaviour is robust within a wide magnetic field range up to 12 K above T N . Solid lines are guides for the eyes. Inset shows the same plot at H > H c . The T 2 behaviour is satisfied when the magnetic field is close to H c , but deviates quickly as an anomaly in ε is observable at higher magnetic fields. Full size image In the absence of spin anisotropy, the induced magnon gap from Zeeman energy can be calculated as Δ= gμ B ( H − H c )Δ S . Using the g -factor value ( g zz =2.1) reported in a far infrared spectroscopy work [29] , we obtain Δ=11.2 K, which is smaller than the fitted value Δ=14.7±1.1 K from the ε data at 45 T. This discrepancy seems to decrease once the effect of spin anisotropy is taken into account (see Supplementary Fig. 5 and Supplementary Note 4 for details). Non-classical behaviour in dielectric constant in a broad field and temperature window For a classical FE or AF system, one expects a Curie-law behaviour, that is, linear dependence of inverse susceptibility on T . However, we find that the inverse dielectric constant follows a quadratic dependence on temperature in a broad field and temperature window. Figure 3b shows ( ε − ε 0 ) −1 as a function of ( T − T N ) 2 , demonstrating the quadratic dependence that can be observed as high as 12 K above T N around H c (also see Supplementary Fig. 6 and Supplementary Note 5 for details). The quadratic dependence is also robust in a wide range of fields, that is, between 9 and 38 T, showing that the non-classical behaviour manifests itself in a wide region of the H – T phase diagram due to quantum fluctuations. Phase diagram alluding the magnetic QPT All T - and H -dependent experiments are summarized in the H–T phase diagram ( Fig. 4 ). The resultant phase boundaries resemble archetypal phase boundaries for a continuous QPT, namely, the V-shaped quantum critical region between two different phases [1] , [2] , [3] , [7] , [39] . The AF order appears below T N =6.7 K at H =0 and is continuously suppressed to T =0 by the c -axis magnetic field at H c =37.1 T. M saturates above H c and a gapped spin-polarized state develops with a characteristic energy scale that is observed by the dielectric constant measurement. 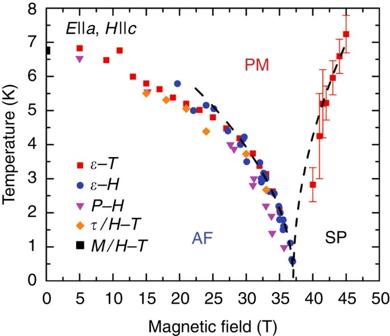Figure 4:H−Tphase diagram of Ba2CoGe2O7. AF to PM phase boundary is marked by peaks inε(T),ε(H),dP(H)/dH, anomalies inτ/HversusTand direct current magnetic susceptibility (M/H) data (red squares, blue circles, purple triangles, orange diamonds, and black square, respectively). The crossover between field-induced quantum critical to gapped spin-polarized state atH>Hcis indicated by anomalies inε(T) (T*, red squares aboveHcsee text). Dashed lines below and aboveHcshow the fit to the equationTN∝|H−Hc|1/2andT*∝|H−Hc|1/2, respectively. Figure 4: H − T phase diagram of Ba 2 CoGe 2 O 7 . AF to PM phase boundary is marked by peaks in ε ( T ), ε ( H ), dP ( H )/ dH , anomalies in τ / H versus T and direct current magnetic susceptibility ( M / H ) data (red squares, blue circles, purple triangles, orange diamonds, and black square, respectively). The crossover between field-induced quantum critical to gapped spin-polarized state at H > H c is indicated by anomalies in ε ( T ) ( T *, red squares above H c see text). Dashed lines below and above H c show the fit to the equation T N ∝ | H − H c | 1/2 and T * ∝ | H − H c | 1/2 , respectively. Full size image To understand the link between FE and AF in BCGO, we construct a phenomenological GL free energy based on the pd H model. Based on the analyses of the GL model, we found that the alternating distortion of CoO 4 tetrahedra along the [110] direction ( Fig. 1a ) plays a key role in realizing the linear coupling term that is proportional to λ sin2 κ · P y L x M in the free energy ( x- and y -directions refers to the [110] and [ ] directions in the tetragonal setting, respectively). Ultimately, through this coupling, we find a linear relation between the magnetic contribution to the dielectric constant and the AF susceptibility χ L ( Supplementary Note 4 ): where M S is the saturation value of the magnetization, ε 0 is the lattice contribution to the dielectric constant ( ε → ε 0 for T >> T N ), and λ is the ME coupling coefficient. The proportionality between ε − ε 0 and χ L qualitatively explains the occurrence of a peak in ε ( T ) at the AF phase transition and the increase of ε on cooling due to enhanced fluctuations of L near T =0 ( Supplementary Note 4 ). This relation is especially useful for studying the AF susceptibility when L is almost suppressed to 0 (that is, when M is nearly saturated by the applied magnetic field). We note that fluctuations of the AF order parameter usually do not affect the dielectric constant and can only be measured with tools that can detect excitations on the zone boundary, such as neutron scattering. It is then worth discussing the implications of the dielectric properties, for example, characteristic power law, in relation to the AF QCP. Earlier studies of BCGO suggested a tetragonal crystal symmetry, and thus the fourfold or U (1) symmetry for describing the in-plane magnetization [26] , [28] . However, recent detailed investigations indeed revealed the presence of the twofold magnetization in the plane and an orthorhombic Cm ′ m 2′ magnetic space group [30] , [31] . The twofold symmetry is likely to be reinforced by the small but unavoidable in-plane magnetic field component, coming from the tilting of the magnetic field from the c -axis. Therefore, the proper effective theory close to the QCP should become the Ising model, which predicts an effective dimension = d + z =4, where d is the spatial dimension of the system ( d =3) and z =1 the dynamical exponent. On the other hand, a U (1) symmetric model would lead to a QCP that belongs to the BEC universality class, of which dynamic exponent is z =2. It is noted that at least three experimental observations are supportive of the scenario of a dynamical exponent z =1. The first observation is the measured field dependence of T N near the QCP: T N ∝ | H − H c | 1/2 ( Fig. 4 and Supplementary Fig. 5a ). This should be contrasted with the T N ∝ | H − H c | 2/3 dependence that would be obtained for a BEC-QCP in d =3. The second observation is that a linear extrapolation of the measured spin gap at high fields crosses the T =0 line at a magnetic field value, which is significantly lower than H c ( Supplementary Fig. 5b ). Because Δ ∝ | H − H c | zν and ν =1/2, this observation is again consistent with z =1 and not with z =2. Finally, according to equation (3), (ε−ε 0 ) ∝ χ L ∝ T −(2− η )/ z = T −2 for d =3 and z =1 (up to logarithmic corrections), in agreement with our observations (see Fig. 3b ). In contrast, ε − ε 0 ∝ χ L ∝ 1/ T 3/2 for a d =3 BEC-QCP. Thus, = d + z =4 is equal to the upper critical dimension, justifying the mean-field GL description that we used to derive equation (3). The observation of AF quantum fluctuations by means of intrinsic ME coupling in BCGO opens a new pathway to study coupled orders in condensed matter physics. Enhancement of ε at the magnetic field-induced phase transition close to T =0, and its non-classical power-law behaviour in an insulating magnet present an interesting counterpart to the non-Fermi-liquid behaviour found near a magnetic QCP in metallic systems [2] , [3] . It should be noted that this phenomena can be observed in other multiferroics with a similar structural staggering feature for the relevant magnetic ions. Therefore, the discovery provided here prompts further investigations to search for this novel possibility in other systems and reflects the extreme versatility of the multiferroic phenomena, even at the quantum mechanical level. Sample synthesis Single crystalline samples were grown using the floating zone method. The feed rods for the floating zone method were prepared by a solid-state reaction method in air. Measurement of FE properties For dielectric constant and electric polarization measurements, electrical contacts were made by using silver epoxy on both sides of rectangular thin platelet samples. Dielectric constants were measured using capacitance bridges (GR1615A, General Radio and AH2700A, Andeen–Hagerling). ε ( H ) curve at different frequencies (0.2, 2 and 2 kHz) was measured using AH2700A. Electric polarization was obtained by integrating the pyro- and magneto-electric currents using an electrometer (KE617, Keithley). P ( T ) or P ( H ) curves were obtained after poling samples from ~30 K down to the measuring temperature in a static poling electric field of 300 kV m −1 . To obtain accurate T values for the polarization and dielectric constant measurements in high magnetic fields, we pre-calibrated a capacitance sensor (Lakeshore) at zero field between 0.5 and 30 K prior to the measurement and used it in a finite magnetic field. We maintained the temperature below 30 K until the experiment was completed to avoid thermal hysteresis in the capacitance sensor. Measurement of magnetic properties Torque signals were measured using a capacitive cantilever made of BeCu foil. For torque measurements, a Cernox sensor (Lakeshore), without magnetic field correction, was used. Magnetization curves were measured using a pickup-coil/extraction magnetometer in a short pulse magnet at NHMFL-LANL, Los Alamos. These data were calibrated against the absolute value found using a vibrating sample magnetometer (PPMS-9, Quantum Design). All direct current high magnetic field measurements were performed using either a resistive magnet (≤35 T) or a hybrid magnet (11 T≤ H ≤45 T) at NHMFL, Tallahassee. How to cite this article: Kim, J. W. et al. Manifestation of magnetic quantum fluctuations in the dielectric properties. Nat. Commun. 5:4419 doi: 10.1038/ncomms5419 (2014).